APF lncRNA regulates autophagy and myocardial infarction by targeting miR-188-3p The abnormal autophagy is associated with a variety of cardiovascular diseases. Long noncoding RNAs (lncRNAs) are emerging as new factors in gene regulation, but how lncRNAs operate in the regulation of autophagy in the heart is unclear. Here we report that a long noncoding RNA, named autophagy promoting factor (APF), can regulate autophagic cell death by targeting miR-188-3p and ATG7. The results show that miR-188-3p suppresses autophagy and myocardial infarction by targeting ATG7. Further, we find that APF lncRNA regulates miR-188-3p, and thus affects ATG7 expression, autophagic cell death and myocardial infarction. Our present study reveals a novel regulating model of autophagic programme, which comprises APF, miR-188-3p and ATG7 in the heart. Modulation of their levels may serve as potential targets and diagnostic tools for novel therapeutic strategies of myocardial infarction and heart failure. Autophagy is an evolutionarily conserved process in response to stress. During autophagy, bulk cellular components like abnormal protein aggregates and damaged organelles are sequestered into lysosomes and degraded [1] , [2] . The abnormal autophagy is related to a variety of pathological disorders including cancer, neurodegenerative and cardiovascular diseases [3] , [4] , [5] , [6] . Autophagy involves a set of Atg genes that are conserved from yeast to human. ATG7 encodes the only one E1 enzyme in autophagy system and has a critical role in membrane elongation. ATG7 is not only an important marker of autophagy, but also a key autophagy promoter that functions in the regulation of cell death and survival [7] . Being a key autophagy-promoting gene, ATG7 is involved in numerous diseases, including cancer, cardiovascular and neurological diseases [8] , [9] , [10] . Although ATG7 plays an important role in cell survival/death determination and disease progression, the molecular regulation of ATG7 during stress response in cardiomyocytes remains to be elucidated. MicroRNAs (miRNAs) are endogenous short noncoding RNA molecules with 22–24 nucleotides. Through binding to targeted mRNA, miRNAs are able to affect the stability and translation of mRNAs. MiRNAs participate in the regulation of a variety of cellular events such as apoptosis, proliferation, development, differentiation and cell conversion. Several miRNAs are related to autophagy. MiR-18a induces autophagic cell death in colon cancer cells [11] . MiR-155 promotes autophagy in macrophages [12] . MiR-30a regulates autophagy by targeting to beclin1 in cancer cell [13] . However, it remains largely unknown as to how autophagy is regulated by miRNAs in cardiomyocytes. Long non-coding RNAs (lncRNAs) are a set of RNAs longer than 200nt. LncRNAs participate in various cellular processes, including genomic imprinting, cell fate determination, RNA alternative splice and chromatin modification, and is important for development, differentiation and metabolism [14] . Also, lncRNAs are involved in lots of human diseases. The study of lncRNAs function in cardiac diseases has only just begun. LncRNAs have been identified in cardiomyocytes and are essential for heart development. Fendrr and Braveheart are two lncRNAs that play an important role in cardiomyocyte differentiation [15] , [16] . However, whether lncRNA participates in the regulation of cardiomyocyte autophagy remains unknown. Our present work reveals that ATG7 is a target of miR-188-3p and miR-188-3p participates in the suppression of ATG7 translation. MiR-188-3p inhibits autophagy and cell death through targeting ATG7 in vivo and in vitro . Moreover, our study further suggests that a long noncoding RNA, autophagy-promoting factor (APF), directly binds to miR-188-3p and therefore inhibits its activity. APF regulates ATG7 expression and the consequent cardiac autophagy through miR-188-3p. In short, APF regulates autophagic programme and autophagic cell death through targeting the miR-188-3p/ATG7 pathway. Our data shed new light on the understanding of the interaction between lncRNA and miRNA in molecular regulation of autophagic programme and myocardial infarction. miR-188-3p participates in the regulation of ATG7 expression ATG7 is a key autophagy promoting gene, which is involved in ischaemia/reperfusion (I/R)-induced myocardial injury ( Supplementary Fig. 1a,b ). MiRNAs are a class of small non-coding RNAs and act as negative regulators of gene expression. To explore whether ATG7 could be regulated by miRNA, we first analysed the 3′UTR of ATG7 using the RNAhybrid programme and found several potential miRNA-binding sites. To identify which miRNA was involved in the regulation of ATG7, we employed immunoblot to detect ATG7 levels. Among several miRNAs, miR-188-3p significantly reduced the levels of ATG7 ( Fig. 1a,b ), which promoted us to focus on its function. We first tested whether knockdown of miR-188-3p could alter the expression of endogenous ATG7. Our results showed that knockdown of endogenous miR-188-3p by antagomir induced an increase in ATG7 expression ( Fig. 1c ). Anoxia/reoxygenation (A/R), which had been reported to induce autophagy, resulted in an increase in ATG7 expression, while enforced expression of miR-188-3p inhibited the increase of ATG7 expression levels on A/R ( Fig. 1d ). To understand whether the effect of miR-188-3p on ATG7 was specific, we then employed the target protector technology [17] . The inhibitory effect of miR-188-3p on ATG7 expression was reduced in the presence of the target protector ( Fig. 1e ). ATG7 upregulation was attenuated by the target protector in response to A/R ( Fig. 1f ). Beclin 1 is a well-known key regulator of autophagy [18] , [19] . Recent study has shown that Beclin 1 mediates the autophagic cell death in cardiomyocytes [20] . Thus, we also tested whether Beclin 1 could be regulated by miR-188-3p. Our results showed that miR-188-3p had no effect on Beclin 1 ( Supplementary Fig. 1c,d ), indicating that miR-188-3p could specifically regulate ATG7. 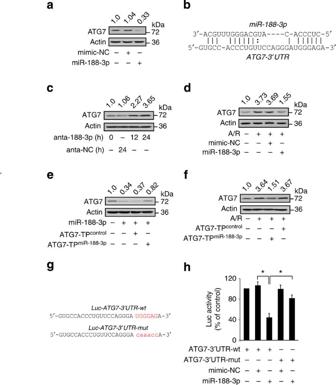Figure 1: miR-188-3p participates in the regulation of ATG7 expression. (a) miR-188-3p suppresses the expression of ATG7. Cardiomyocytes were transfected with mimic-miR-188-3p (miR-188-3p) or mimic negative control (mimic-NC). The levels of ATG7 were analysed by immunoblot.n=3. (b) Putative miR-188-3p binding site in the 3′UTR region of ATG7. (c) Knockdown of miR-188-3p increases the expression levels of ATG7. Cardiomyocytes were transfected with miR-188-3p antagomir (anta-188-3p) or the antagomir-negative control (anta-NC), the levels of ATG7 were analysed by immunoblot;n=3. (d) miR-188-3p attenuates the increase in ATG7 levels on A/R. Cardiomyocytes were transfected with miR-188-3p or the mimic-NC, and then exposed to A/R. The levels of ATG7 were analysed by immunoblot;n=3. (e) ATG7 target protector attenuates the reduction of ATG7 induced by miR-188-3p. Cardiomyocytes were transfected with the ATG7 target protector (ATG7-TPmiR-188-3p) or the control (ATG7-TPcontrol). ATG7 levels were detected by immunoblot;n=3. (f) ATG7 target protector inhibits A/R-induced ATG7 upregulation. Cardiomyocytes were transfected with the ATG7-TPmiR-188-3por ATG7-TPcontrol, and then exposed to A/R. The levels of ATG7 were analysed by immunoblot;n=3. (g) ATG7 wild-type (WT) 3′UTR and a mutated 3′UTR in the miR-188-3p-binding site are shown. (h) miR-188-3p suppresses ATG7 translation. HEK293 cells were transfected with miR-188-3p, mimic-NC, the luciferase constructs of the wild-type ATG7-3′UTR (ATG7-3’UTR-wt) or a mutated ATG7-3′UTR (ATG7-3′UTR-mut). The luciferase activity was analysed. Data are shown as mean±s.e.m. of three independent experiments. *P<0.05 in one-way analysis of variance. Figure 1: miR-188-3p participates in the regulation of ATG7 expression. ( a ) miR-188-3p suppresses the expression of ATG7. Cardiomyocytes were transfected with mimic-miR-188-3p (miR-188-3p) or mimic negative control (mimic-NC). The levels of ATG7 were analysed by immunoblot. n =3. ( b ) Putative miR-188-3p binding site in the 3′UTR region of ATG7. ( c ) Knockdown of miR-188-3p increases the expression levels of ATG7. Cardiomyocytes were transfected with miR-188-3p antagomir (anta-188-3p) or the antagomir-negative control (anta-NC), the levels of ATG7 were analysed by immunoblot; n =3. ( d ) miR-188-3p attenuates the increase in ATG7 levels on A/R. Cardiomyocytes were transfected with miR-188-3p or the mimic-NC, and then exposed to A/R. The levels of ATG7 were analysed by immunoblot; n =3. ( e ) ATG7 target protector attenuates the reduction of ATG7 induced by miR-188-3p. Cardiomyocytes were transfected with the ATG7 target protector (ATG7-TP miR-188-3p ) or the control (ATG7-TP control ). ATG7 levels were detected by immunoblot; n =3. ( f ) ATG7 target protector inhibits A/R-induced ATG7 upregulation. Cardiomyocytes were transfected with the ATG7-TP miR-188-3p or ATG7-TP control , and then exposed to A/R. The levels of ATG7 were analysed by immunoblot; n =3. ( g ) ATG7 wild-type (WT) 3′UTR and a mutated 3′UTR in the miR-188-3p-binding site are shown. ( h ) miR-188-3p suppresses ATG7 translation. HEK293 cells were transfected with miR-188-3p, mimic-NC, the luciferase constructs of the wild-type ATG7-3′UTR (ATG7-3’UTR-wt) or a mutated ATG7-3′UTR (ATG7-3′UTR-mut). The luciferase activity was analysed. Data are shown as mean±s.e.m. of three independent experiments. * P <0.05 in one-way analysis of variance. Full size image We employed the luciferase assay system to test whether miR-188-3p could influence the translation of ATG7. As shown in Fig. 1h , the luciferase reporter assay revealed that the wild-type 3′-UTR of ATG7 exhibited a low translation level in the presence of miR-188-3p, whereas the mutated 3′-UTR ( Fig. 1g ) did not show a significant response to miR-188-3p. Taken together, these data suggest that ATG7 is a specific target of miR-188-3p. miR-188-3p inhibits autophagy and cell death in vitro and in vivo We attempted to understand the role of miR-188-3p in autophagy under the pathological condition, and observed that A/R reduced the levels of miR-188-3p ( Fig. 2a ). LC3-II relocalizes to the autophagosomal membranes during autophagy. Thus, the accumulation of GFP-LC3 puncta provides an effective way to detect autophagosomes. We found that A/R induced an increased GFP-LC3 punctuate structures, whereas enforced expression of miR-188-3p significantly reduced punctate accumulations of GFP-LC3 ( Fig. 2b ). In addition, miR-188-3p also induced a reduction in LC3-II expression levels on A/R treatment ( Fig. 2c ). The results of an EM analysis showed that miR-188-3p reduced autophagic vesicles in cardiomyocytes ( Fig. 2d ). Also, enforced expression of miR-188-3p significantly reduced cell death induced by A/R ( Fig. 2e ). Taken together, these results suggest that miR-188-3p inhibits autophagy and cell death induced by A/R in cardiomyocytes. 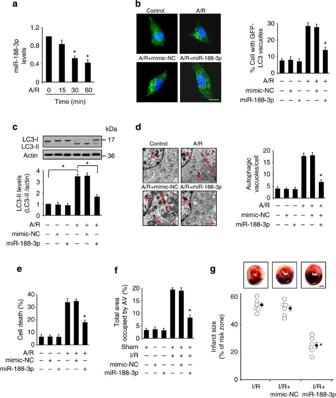Figure 2: miR-188-3p inhibits autophagy under the pathological condition. (a) Cardiomyocytes were exposed to A/R and miR-188-3p levels were analysed by qRT-PCR. Data are shown as mean±s.e.m. of four independent experiments. *P<0.05 versus control in Student’st-test. (b) miR-188-3p inhibits punctate accumulations of GFP-LC3 induced by A/R. Cardiomyocytes were treated with adenoviral GFP-LC3, miR-188-3p and mimic-NC, and cells were exposed to A/R. Representative photos of GFP-LC3 cells were shown in the left panel, and the percentage of cells with GFP-LC3 puncta was quantified in the right panel. Data are shown as mean±s.e.m. of three independent experiments. *P<0.05 versus A/R alone in one-way analysis of variance. Scale bar, 20 μm. (c) Representative immunoblot for conversion of LC3-I to LC3-II. Cardiomyocytes were treated as described in (b). The positions of LC3-I and LC3-II are indicated. The densitometric analysis of western blot of LC3-II is shown (lower panel). *P<0.05. (d,e) Cardiomyocytes were treated as described in (b). Representative EM images and quantification of autophagic vacuoles was shown in (d). Scale bar, 500 nm. The arrows depict autophagosomes, and the nucleus is denoted byN. Data are shown as mean±s.e.m. of three independent experiments. *P<0.05 versus A/R alone in one-way analysis of variance. Quantfication of cell death is shown in (e). Data are shown as mean±s.e.m. of three independent experiments. *P<0.05 versus A/R alone in one-way analysis of variance. (f) Mice were injected with miR-188-3p or mimic-NC as described in methods, and then were subjected to 45 min ischaemia and 3 h reperfusion. Quantification of autophagic vacuoles was shown. Data are shown as mean±s.e.m. of six independent experiments. *P<0.05 versus I/R alone in one-way analysis of variance. (g) Mice were treated as described in (f). Hearts were sliced, stained with TTC and fixed to delineate live (red) from dead or infarcted tissue (white). Infarcts were quantified by planimetry and expressed as a percentage of risk zone. Images above the graph show representative slices from each group (bar=2 mm). Open circles represent individual data points and closed circles represent means with s.e.m. (n=6 all groups). *P<0.05 versus I/R alone. Figure 2: miR-188-3p inhibits autophagy under the pathological condition. ( a ) Cardiomyocytes were exposed to A/R and miR-188-3p levels were analysed by qRT-PCR. Data are shown as mean±s.e.m. of four independent experiments. * P <0.05 versus control in Student’s t- test. ( b ) miR-188-3p inhibits punctate accumulations of GFP-LC3 induced by A/R. Cardiomyocytes were treated with adenoviral GFP-LC3, miR-188-3p and mimic-NC, and cells were exposed to A/R. Representative photos of GFP-LC3 cells were shown in the left panel, and the percentage of cells with GFP-LC3 puncta was quantified in the right panel. Data are shown as mean±s.e.m. of three independent experiments. * P <0.05 versus A/R alone in one-way analysis of variance. Scale bar, 20 μm. ( c ) Representative immunoblot for conversion of LC3-I to LC3-II. Cardiomyocytes were treated as described in ( b ). The positions of LC3-I and LC3-II are indicated. The densitometric analysis of western blot of LC3-II is shown (lower panel). * P <0.05. ( d , e ) Cardiomyocytes were treated as described in ( b ). Representative EM images and quantification of autophagic vacuoles was shown in ( d ). Scale bar, 500 nm. The arrows depict autophagosomes, and the nucleus is denoted by N . Data are shown as mean±s.e.m. of three independent experiments. * P <0.05 versus A/R alone in one-way analysis of variance. Quantfication of cell death is shown in ( e ). Data are shown as mean±s.e.m. of three independent experiments. * P <0.05 versus A/R alone in one-way analysis of variance. ( f ) Mice were injected with miR-188-3p or mimic-NC as described in methods, and then were subjected to 45 min ischaemia and 3 h reperfusion. Quantification of autophagic vacuoles was shown. Data are shown as mean±s.e.m. of six independent experiments. * P <0.05 versus I/R alone in one-way analysis of variance. ( g ) Mice were treated as described in ( f ). Hearts were sliced, stained with TTC and fixed to delineate live (red) from dead or infarcted tissue (white). Infarcts were quantified by planimetry and expressed as a percentage of risk zone. Images above the graph show representative slices from each group (bar=2 mm). Open circles represent individual data points and closed circles represent means with s.e.m. ( n =6 all groups). * P <0.05 versus I/R alone. Full size image We tested whether miR-188-3p played a role in the pathogenesis of myocardial infarction in the animal model. We employed the myocardial I/R model and found that I/R induced a reduction in miR-188-3p levels ( Supplementary Fig. 2a ). However, enforced expression of miR-188-3p in vivo resulted in a reduction in ATG7 levels on I/R injury ( Supplementary Fig. 2b ). Administration of the target protector technology in vivo showed that I/R-induced ATG7 expression was attenuated in the presence of ATG7 target protector ( Supplementary Fig. 2c ). These results indicated that ATG7 was indeed regulated by miR-188-3p in vivo . We further demonstrated that enforced expression of miR-188-3p in vivo attenuated autophagy ( Fig. 2f ) and myocardial infarction sizes ( Fig. 2g ) in response to I/R injury. Moreover, ATG7 overexpression ( Supplementary Fig. 3a,b ) abolished the inhibitory effect of miR-188-3p on infarct sizes ( Supplementary Fig. 3c ). In addition, we also analysed the effects of miR-188-3p in border zone and remote zone, given that three zones have vastly divergent biology in infarcted myocardium. The results indicated that miR-188-3p had no effect on the border zone ( Supplementary Fig. 3d ) and the remote zone ( Supplementary Fig. 3e ). Taken together, these data suggest that miR-188-3p is able to inhibit autophagy and autophagic cell death in the heart. APF is able to directly bind to miR-188-3p and regulate miR-188-3p activity We explored the underlying mechanism responsible for miR-188-3p downregulation in response to A/R treatment. We first tested whether lncRNA, which had been reported to act as endogenous sponge RNA to interact with miRNAs [21] , [22] , [23] , could be involved in the autophagic pathway of A/R treatment. We screened some lncRNAs in the heart from a result of lncRNA array performed by Fantom company. We carried out qRT–PCR to detect lncRNAs levels on A/R treatment. Among those lncRNAs, only AK079427, which we named APF, was significantly upregulated on A/R treatment ( Fig. 3a ). APF is 1,695-nt long and it is polyadenylated. The full-length of APF is poorly conserved across species, but it is conserved between species in the binding site of miR-188-3p ( Supplementary Fig. 4a ). The expression level of APF is more than one-third of the miR-188-3p in the mouse heart ( Supplementary Fig. 4b ). APF and miR-188-3p have similar expression pattern in cells ( Supplementary Fig. 4c,d ) and tissues ( Supplementary Fig. 4e,f ). To understand whether APF could interact with miR-188-3p in the autophagic pathway, we compared the sequences of APF with that of miR-188-3p using the bioinformatics programme RNAhybrid and noticed that APF contained a binding site of miR-188-3p ( Fig. 3b ). Next, we produced a luciferase construct of APF (Luc-APF-wt) and a mutated form (Luc-APF-mut) ( Fig. 3c ). Luciferase assay revealed that miR-188-3p could suppress the luciferase activity of APF, but it had less effect on the mutated form of APF ( Fig. 3c ). These results revealed that APF may interact with miR-188-3p by this putative binding site. 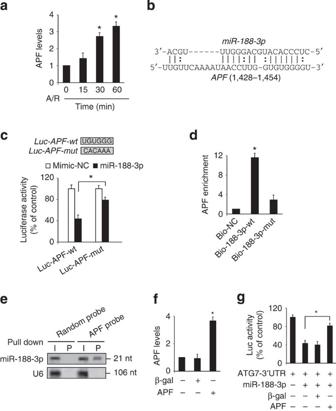Figure 3: The interaction between APF and miR-188-3p. (a) APF expression levels on treatment with A/R. Cardiomyocytes were treated with A/R. APF expression levels were analysed by qRT-PCR. Data are shown as mean±s.e.m. of three independent experiments. *P<0.05 versus control in Student’st-test. (b) APF RNA contains a site complementary to miR-188-3p. (c) Luciferase assay. MiR-188-3p-binding site in the APF RNA wild-type form (Luc-APF-wt) and the mutated form (Luc-APF-mut) are shown in the upper panel. HEK293 cells were transfected with miR-188-3p or mimic-NC, then transfected with the luciferase constructs of Luc-APF-wt or Luc-APF-mut. The luciferase activity was analysed. Data are shown as mean±s.e.m. of three independent experiments. *P<0.05 in one-way analysis of variance. (d) miR-188-3p can bind directly to APFin vivo. Cardiomyocytes were transfected with biotinylated wild-type miR-188-3p (Bio-188-3p-wt) or biotinylated mutant miR-188-3p (Bio-188-3p-mut). A biotinylated miRNA that is not complementary to APF was used as a negative control (Bio-NC). Forty-eight hours after transfection, cells were harvested for biotin-based pull-down assay. APF expression levels were analysed by real-time PCR. Data are shown as mean±s.e.m. of four independent experiments. *P<0.05 versus Bio-NC in one-way analysis of variance. (e) APF can bind to miR-188-3pin vivo. Cardiomyocyte lysates were incubated with APF probe or random probe-coated magnetic bead. After washing and enrichment of beads/RNA complex, RNA was eluted from the streptavidin beads and was analysed by northern blot. I, input (10% samples were loaded); P, pellet (100% samples were loaded). (f) Enforced expression of APF increases the expression levels of APF. Cardiomyocytes were infected with adenoviral APF or β-gal. Twenty-four hours after infection, APF levels were analysed by real-time PCR. Data are shown as mean±s.e.m. of three independent experiments. *P<0.05 versus control in one-way analysis of variance. (g) APF inhibits miR-188-3p activity. Cardiomyocytes were infected with adenoviral APF or β-gal, then transfected with miR-188-3p and ATG7-3′UTR. Luciferase activity was analysed. Data are shown as mean±s.e.m. of four independent experiments. *P<0.05 in one-way analysis of variance. Figure 3: The interaction between APF and miR-188-3p. ( a ) APF expression levels on treatment with A/R. Cardiomyocytes were treated with A/R. APF expression levels were analysed by qRT-PCR. Data are shown as mean±s.e.m. of three independent experiments. * P <0.05 versus control in Student’s t- test. ( b ) APF RNA contains a site complementary to miR-188-3p. ( c ) Luciferase assay. MiR-188-3p-binding site in the APF RNA wild-type form (Luc-APF-wt) and the mutated form (Luc-APF-mut) are shown in the upper panel. HEK293 cells were transfected with miR-188-3p or mimic-NC, then transfected with the luciferase constructs of Luc-APF-wt or Luc-APF-mut. The luciferase activity was analysed. Data are shown as mean±s.e.m. of three independent experiments. * P <0.05 in one-way analysis of variance. ( d ) miR-188-3p can bind directly to APF in vivo . Cardiomyocytes were transfected with biotinylated wild-type miR-188-3p (Bio-188-3p-wt) or biotinylated mutant miR-188-3p (Bio-188-3p-mut). A biotinylated miRNA that is not complementary to APF was used as a negative control (Bio-NC). Forty-eight hours after transfection, cells were harvested for biotin-based pull-down assay. APF expression levels were analysed by real-time PCR. Data are shown as mean±s.e.m. of four independent experiments. * P <0.05 versus Bio-NC in one-way analysis of variance. ( e ) APF can bind to miR-188-3p in vivo . Cardiomyocyte lysates were incubated with APF probe or random probe-coated magnetic bead. After washing and enrichment of beads/RNA complex, RNA was eluted from the streptavidin beads and was analysed by northern blot. I, input (10% samples were loaded); P, pellet (100% samples were loaded). ( f ) Enforced expression of APF increases the expression levels of APF. Cardiomyocytes were infected with adenoviral APF or β-gal. Twenty-four hours after infection, APF levels were analysed by real-time PCR. Data are shown as mean±s.e.m. of three independent experiments. * P <0.05 versus control in one-way analysis of variance. ( g ) APF inhibits miR-188-3p activity. Cardiomyocytes were infected with adenoviral APF or β-gal, then transfected with miR-188-3p and ATG7-3′UTR. Luciferase activity was analysed. Data are shown as mean±s.e.m. of four independent experiments. * P <0.05 in one-way analysis of variance. Full size image Further, we tested whether APF could directly bind to miR-188-3p in vivo . We applied a biotin–avidin pull-down system to test whether miR-188-3p could pull down APF. Cardiomyocytes were transfected with biotinylated miR-188-3p, then harvested for biotin-based pull-down assay. APF was pulled down and analysed by qRT-PCR. The introduction of mutations that disrupt base pairing between APF and miR-188-3p led to the inability of miR-188-3p to pull down APF ( Fig. 3d ), indicating that miR-188-3p recognizes APF in a sequence-specific manner. We also employed inverse pull-down assay to test whether APF could pull down miR-188-3p using biotin-labelled-specific APF probe. MiR-188-3p was co-precipitated and analysed by northern blot ( Fig. 3e ). Further, we detected the subcellular location of APF and miR-188-3p. It showed that APF was expressed both in the nucleus and cytoplasm, while miR-188-3p was mainly expressed in the cytoplasm ( Supplementary Fig. 5a ). Thus, we applied the biotin-labelled-specific APF probe to assay where the interaction between APF and miR-188-3p occurred. The results showed that miR-188-3p could be co-precipitated in the cytoplasm, but not in the nucleus ( Supplementary Fig. 5b,c ). Finally, we tested whether APF could affect the activity of miR-188-3p. The luciferase activity analysis showed that enforced expression of APF ( Fig. 3f ) counteracted the inhibitory effect of miR-188-3p ( Fig. 3g ), whereas the mutant APF had no effect on miR-188-3p ( Supplementary Fig. 5d ), suggesting that APF inhibited the activity of miR-188-3p. Taken together, these data suggest that APF is able to directly bind to miR-188-3p and regulate its activity. APF conveys the autophagic signal in cardiomyocytes We tested whether APF played a functional role in autophagy. In cardiomyocytes, knockdown of APF by an siRNA technology effectively reduced the expression of APF ( Fig. 4a ). Further, knockdown of APF ( Supplementary Fig. 6a ) reduced LC3-II levels ( Fig. 4b ) and LC3-II punctate accumulations of GFP-LC3 ( Fig. 4c,d ) on A/R treatment. Also, knockdown of APF reduced autophagic vesicles ( Fig. 4e ) and cell death ( Fig. 4f ) on A/R treatment. These results suggest that APF is involved in the regulation of autophagic pathway in cardiomyocytes. 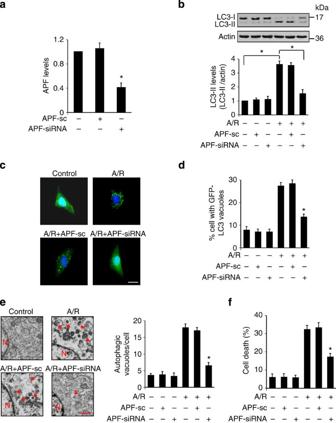Figure 4: APF conveys the autophagic signal in cardiomyocytes. (a) Knockdown of APF by an siRNA technique decreases the expression levels of APF. Cardiomyocytes were infected with adenoviral APF siRNA (APF-siRNA) and its scramble form (APF-sc). Twenty-four hours after infection, APF levels were analysed by real-time PCR. Data are shown as mean±s.e.m. of three independent experiments. *P<0.05 versus control in one-way analysis of variance. (b) Knockdown of APF inhibits the conversion of LC3-I to LC3-II in response to A/R. Cardiomyocytes were infected with adenoviral APF-siRNA or APF-sc. Twenty-four hours after infection, cells were treated with A/R. Representative immunoblot for conversion of LC3-I to LC3-II was shown. The densitometric analysis of western blot of LC3-II is shown (lower panel). *P<0.05. (c,d) Knockdown of APF inhibits punctate accumulations of GFP-LC3. Cardiomyocytes were infected with adenoviral GFP-LC3, APF-siRNA or APF-sc. Twenty-four hours, after infection cells were treated with A/R. Representative images show GFP-LC3 staining (c), Scale bar, 20 μm. The percentage of cells with GFP-LC3 puncta was quantified in (d). Data are shown as mean±s.e.m. of four independent experiments. *P<0.05 versus A/R alone in one-way analysis of variance. (e,f) Knockdown of APF reduces autophagic vacuoles and cell death. Cardiomyocytes were treated as described in (b). Quantification of autophagic vacuoles was shown in (e). Quantification of cell death was shown in (f). Data are shown as mean±s.e.m. of four independent experiments. *P<0.05 versus A/R alone in one-way analysis of variance. Figure 4: APF conveys the autophagic signal in cardiomyocytes. ( a ) Knockdown of APF by an siRNA technique decreases the expression levels of APF. Cardiomyocytes were infected with adenoviral APF siRNA (APF-siRNA) and its scramble form (APF-sc). Twenty-four hours after infection, APF levels were analysed by real-time PCR. Data are shown as mean±s.e.m. of three independent experiments. * P <0.05 versus control in one-way analysis of variance. ( b ) Knockdown of APF inhibits the conversion of LC3-I to LC3-II in response to A/R. Cardiomyocytes were infected with adenoviral APF-siRNA or APF-sc. Twenty-four hours after infection, cells were treated with A/R. Representative immunoblot for conversion of LC3-I to LC3-II was shown. The densitometric analysis of western blot of LC3-II is shown (lower panel). * P <0.05. ( c , d ) Knockdown of APF inhibits punctate accumulations of GFP-LC3. Cardiomyocytes were infected with adenoviral GFP-LC3, APF-siRNA or APF-sc. Twenty-four hours, after infection cells were treated with A/R. Representative images show GFP-LC3 staining ( c ), Scale bar, 20 μm. The percentage of cells with GFP-LC3 puncta was quantified in ( d ). Data are shown as mean±s.e.m. of four independent experiments. * P <0.05 versus A/R alone in one-way analysis of variance. ( e , f ) Knockdown of APF reduces autophagic vacuoles and cell death. Cardiomyocytes were treated as described in ( b ). Quantification of autophagic vacuoles was shown in ( e ). Quantification of cell death was shown in ( f ). Data are shown as mean±s.e.m. of four independent experiments. * P <0.05 versus A/R alone in one-way analysis of variance. Full size image APF participates in the autophagic regulation in vivo To understand the role of APF in the pathogenesis of myocardial infarction, we performed I/R injury in the animal model and observed that I/R induced an increase in APF levels ( Supplementary Fig. 6b ). Delivery of adenovirus APF-siRNA in vivo ( Supplementary Fig. 6c ) attenuated autophagy revealed by EM analysis of ventricular tissue ( Fig. 5a ) and LC3-II levels ( Fig. 5b ) on I/R injury. Our results also showed that the mice treated with APF-siRNA exhibited a significant reduction in myocardial infarction sizes in response to I/R injury ( Fig. 5c ), and enforced expression of ATG7 abolished the inhibitory effect of APF knockdown on infarct sizes ( Supplementary Fig. 6d ). Further, we also demonstrated that APF had no effect on the border zone and remote zone ( Supplementary Fig. 6e,f ). In addition, an ameliorated myocardial function was also observed in the mice treated with APF-siRNA on I/R injury ( Fig. 5d ). These data suggest that APF participates in mediating the signal for autophagy and cell death in the heart. 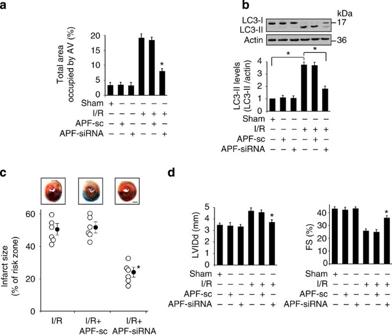Figure 5: APF regulates autophagyin vivo. (a,b) Knockdown of APF reduced autophagy on I/R injury. Mice were injected with adenovirus APF-siRNA or APF-sc as described in methods, then were subjected to 45 min of ischaemia and 3 h of reperfusion (I/R). Quantification of autophagic vacuoles is shown in (a). Data are shown as mean±s.e.m. of six independent experiments. *P<0.05 versus I/R alone in one-way analysis of variance. LC3 levels were analysed by immunoblot (b, upper panel). The densitometric analysis of western blot of LC3-II is shown (lower panel). *P<0.05. (c) Knockdown of APF reduces myocardial infarction on I/Rin vivo. Mice were treated as described in (a). Following IR protocols, hearts were sliced, stained with TTC and fixed to delineate live (red) from dead or infarcted tissue (white). Infarcts were quantified by planimetry and expressed as a percentage of risk zone. Images above the graph show representative slices from each group (scale bar, 2 mm). Open circles represent individual data points and closed circles represent means with s.e.m. (n=6 all groups). *P<0.05 versus I/R alone. (d) Knockdown of APF presents markedly preserved cardiac function after I/R. Mice were injected with adenovirus APF-siRNA or APF-sc as described in Methods, then were subjected to 45 min of ischemia followed by 1 week of reperfusion (I/R). Transthoracic echocardiographic analysis was performed. FS=fractional shortening of left ventricular diameter; LVIDd=diastolic left ventricular internal diameters. Data are shown as mean±s.e.m. of seven independent experiments. *P<0.05 versus I/R alone in one-way analysis of variance. Figure 5: APF regulates autophagy in vivo . ( a , b ) Knockdown of APF reduced autophagy on I/R injury. Mice were injected with adenovirus APF-siRNA or APF-sc as described in methods, then were subjected to 45 min of ischaemia and 3 h of reperfusion (I/R). Quantification of autophagic vacuoles is shown in ( a ). Data are shown as mean±s.e.m. of six independent experiments. * P <0.05 versus I/R alone in one-way analysis of variance. LC3 levels were analysed by immunoblot ( b , upper panel). The densitometric analysis of western blot of LC3-II is shown (lower panel). * P <0.05. ( c ) Knockdown of APF reduces myocardial infarction on I/R in vivo . Mice were treated as described in ( a ). Following IR protocols, hearts were sliced, stained with TTC and fixed to delineate live (red) from dead or infarcted tissue (white). Infarcts were quantified by planimetry and expressed as a percentage of risk zone. Images above the graph show representative slices from each group (scale bar, 2 mm). Open circles represent individual data points and closed circles represent means with s.e.m. ( n =6 all groups). * P <0.05 versus I/R alone. ( d ) Knockdown of APF presents markedly preserved cardiac function after I/R. Mice were injected with adenovirus APF-siRNA or APF-sc as described in Methods, then were subjected to 45 min of ischemia followed by 1 week of reperfusion (I/R). Transthoracic echocardiographic analysis was performed. FS=fractional shortening of left ventricular diameter; LVIDd=diastolic left ventricular internal diameters. Data are shown as mean±s.e.m. of seven independent experiments. * P <0.05 versus I/R alone in one-way analysis of variance. Full size image APF regulates autophagy and cell death through miR-188-3p and ATG7 Since APF interacted with miR-188-3p, we then tested whether APF was able to regulate ATG7, which was the downstream target of miR-188-3p. Knockdown of APF reduced ATG7 expression ( Fig. 6a ). Overexpression of APF resulted in an increase in ATG7 expression levels ( Fig. 6b ). APF but not APF-mut counteracted the inhibitory effect of miR-188-3p on ATG7 expression ( Fig. 6c and Supplementary Fig. 7a ). These results indicate that APF regulates ATG7 expression through miR-188-3p. 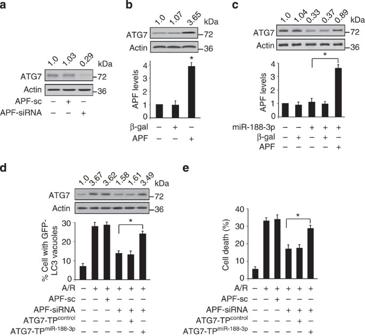Figure 6: APF exerts its autophagic effect through miR-188-3p and ATG7. (a) Knockdown of APF reduces the expression levels of ATG7. Cardiomyocytes were infected with adenoviral APF-siRNA or APF-sc. Twenty-four hours after infection, ATG7 levels were analysed by immunoblot;n=3. (b) Enforced expression of APF induces the increase of ATG7 levels. Cardiomyocytes were infected with adenoviral APF or β-gal. Twenty-four hours after infection, ATG7 levels were analysed by immunoblot (upper panel);n=3. APF levels were analysed by qRT-PCR (lower panel). Data are shown as mean±s.e.m. of three independent experiments. *P<0.05 versus control in one-way analysis of variance. (c) APF reduces the inhibitory effect of miR-188-3p on ATG7 expression. Cardiomyocytes were infected with adenoviral APF or β-gal, and then were transfected with miR-188-3p. ATG7 expression levels were analysed by immunoblot (upper panel);n=4. APF levels were analysed by qRT-PCR (lower panel). Data are shown as mean±s.e.m. of four independent experiments. *P<0.05 in one-way analysis of variance. (d,e) ATG7 target protector attenuates the inhibitory effect of APF knockdown on autophagy induced by A/R. Cardiomyocytes were infected with adenoviral APF-siRNA or APF-sc, transfected with the target protector (ATG7-TPmiR-188-3p) or the control (ATG7-TPcontrol), and then exposed to A/R. ATG7 levels were analysed by immunoblot (d, upper panel);n=3. Autophagy was assessed by GFP-LC3 staining. The percentage of cells with GFP-LC3 puncta was quantified in (d, low panel). Data are shown as mean±s.e.m. of three independent experiments. *P<0.05 in one-way analysis of variance. Quantification of cell death is shown in (e). Data are shown as mean±s.e.m. of three independent experiments. *P<0.05 in one-way analysis of variance. Figure 6: APF exerts its autophagic effect through miR-188-3p and ATG7. ( a ) Knockdown of APF reduces the expression levels of ATG7. Cardiomyocytes were infected with adenoviral APF-siRNA or APF-sc. Twenty-four hours after infection, ATG7 levels were analysed by immunoblot; n =3. ( b ) Enforced expression of APF induces the increase of ATG7 levels. Cardiomyocytes were infected with adenoviral APF or β-gal. Twenty-four hours after infection, ATG7 levels were analysed by immunoblot (upper panel); n =3. APF levels were analysed by qRT-PCR (lower panel). Data are shown as mean±s.e.m. of three independent experiments. * P <0.05 versus control in one-way analysis of variance. ( c ) APF reduces the inhibitory effect of miR-188-3p on ATG7 expression. Cardiomyocytes were infected with adenoviral APF or β-gal, and then were transfected with miR-188-3p. ATG7 expression levels were analysed by immunoblot (upper panel); n =4. APF levels were analysed by qRT-PCR (lower panel). Data are shown as mean±s.e.m. of four independent experiments. * P <0.05 in one-way analysis of variance. ( d , e ) ATG7 target protector attenuates the inhibitory effect of APF knockdown on autophagy induced by A/R. Cardiomyocytes were infected with adenoviral APF-siRNA or APF-sc, transfected with the target protector (ATG7-TP miR-188-3p ) or the control (ATG7-TP control ), and then exposed to A/R. ATG7 levels were analysed by immunoblot ( d , upper panel); n =3. Autophagy was assessed by GFP-LC3 staining. The percentage of cells with GFP-LC3 puncta was quantified in ( d , low panel). Data are shown as mean±s.e.m. of three independent experiments. * P <0.05 in one-way analysis of variance. Quantification of cell death is shown in ( e ). Data are shown as mean±s.e.m. of three independent experiments. * P <0.05 in one-way analysis of variance. Full size image Then, we further tested whether ATG7 is a mediator of APF. To confirm the relationship between APF and ATG7 in autophagic machinery, we knocked down the endogenous APF by APF-siRNA construct ( Supplementary Fig. 7b ), and observed that the inhibitory effect of APF knockdown on ATG7 levels ( Fig. 6d , upper panel), autophagy ( Fig. 6d , low panel) and cell death ( Fig. 6e ) was decreased in the presence of ATG7 target protector. Further experiments showed that ATG7 target protector had no effect on Beclin 1 levels ( Supplementary Fig. 7c ). Taken together, these data suggest that APF targets miR-188-3p/ATG7 axis in the autophagic cascades. An increasing number of studies unveil novel information on autophagy, and our understanding of autophagy in the heart also changes rapidly. It is principally thought that autophagy plays an adaptive role in protecting cardiomyocytes from I/R injury. Upregulation of autophagy in cardiomyocytes is also considered to be an adaptive response to stress, while suppressing the process accelerates heart failure [24] . However, in recent years, emerging evidence has revealed that autophagy is detrimental under certain circumstances. The abnormal autophagy is related to a variety of pathological disorders including cancer, neurodegenerative and cardiovascular diseases [3] , [4] , [5] , [6] . Many studies have revealed that enhanced autophagy contributes to cell death after I/R. Beclin1 RNAi results in enhanced cell survival by reducing I/R-induced autophagy [25] . Impaired autophagosome clearance contributes to cardiomyocyte death in I/R injury [26] . Also, ROS-induced autophagy promotes cell death. I/R injury results in the oxidative stress that enhanced cardiomyocyte autophagy, which further promotes cell apoptosis [27] , [28] . It is also reported that autophagy increases cardiomyocyte death during reperfusion [29] . Moreover, excessive autophagy could destroy a large fraction of organelles and further accentuated pathological death [26] . Consistent with these reports, our work suggests that inhibition of autophagy can protect cell death induced by A/R in cardiomyocytes. In animal model, inhibiting autophagy is also protective for I/R-induced myocardial infarction. Controversy exists in the role of autophagy during I/R. Whether autophagy inhibits or enhances cardiomyocyte death mainly depends on distinct autophagy-related signal pathways triggered by different stimulators with indicated concentration or time. Moreover, more detailed studies are needed to further depict the role of autophagy during myocardial I/R. To date, increasing number of miRNAs are found to be key regulators of different cellular processes, in particular, those related to autophagy [30] . However, few studies identified the regulation mechanism of these miRNAs in cardiomyocytes autophagy. MiR-188-3p is an actively regulated miRNA and is first identified in neuroblastoma cells [31] . It functions in dendritic cells and is crucial for cell differentiation [32] . It is also involved in cardiac remodelling [33] . However, its detailed function in cardiomyocytes and whether it participates in autophagy remain unknown. Moreover, our work here focused on identifying the role of miR-188-3p in regulating autophagy. Our present work finds that miR-188-3p can inhibit autophagic programme and myocardial infarction through targeting ATG7 protein. MiR-188-3p represents a novel mechanism for regulating ATG7 expression and therefore autophagy. LncRNAs have been identified in numerous tissues and cells, like endothelial cell, muscle cell and several cancerous cells [34] , [35] , [36] . LncRNAs have been defined to have important functions in specific cell types, tissues and developmental conditions such as chromatin modification [37] , RNA processing [38] , structural scaffolds [39] and modulation of apoptosis and invasion, and so on [40] . Despite the biological importance of lncRNAs, it is not yet clear whether lncRNAs are involved in the regulation of autophagic programme in the heart. Our present work reveals a novel function of lncRNA participating in regulating autophagy and myocardial infarction. A better understanding of the role of lncRNA in myocardial infarction may yield novel therapeutic target for treating or controlling these diseases. Although the function of lncRNA is important, most of lncRNAs are species specific and represent limited sequence conservation [41] , [42] , [43] , [44] . For example, there is no clear orthologous Bvht, a heart-associated lncRNA, in human or rat genomes [45] , and Bvht represents a lineage-specific nonconserved lncRNA. Moreover, few orthologues of mammalian lncRNAs exist outside of mammals and are highly variable among species [46] , [47] . A large-scale evolutionary study of lncRNA repertoires reveals that many lncRNAs do not show a high interspecies conservation as protein-coding genes [48] . Also, the sequencing analysis of lncRNAs reveals that most of lncRNAs are less conserved [49] . In our study, the full length of APF is also poorly conserved across species, but it is conserved between species in the binding site of miR-188-3p. Thus, the importance of conservation in lncRNAs is greatly questioned, and the less conservation of lncRNAs suggests an essential and irreplaceable role of lncRNAs in biological processes that are fundamental building blocks of life [50] . Generally, lncRNAs are expressed in lower amounts compared with their protein-coding counterparts. However, many lncRNAs maintain important and diverse functions in spite of limited expression levels [51] , [52] , [53] . Thus, it is suggested that low expression level does not hinder the function of lncRNA. In our present study, we found that lncRNA APF affects the activity of miR-188-3p and miR-188-3p downstream target ATG7. Pathological conditions, such as A/R and I/R, induce a significant increase in the APF expression levels, which are sufficient to inhibit miR-188-3p activity and ATG-7 expression, and finally leads to autophagy. It is of note that the lncRNA–miRNA interaction involves many variables, such as RNA–RNA binding energy and the RNA secondary structure [54] , [55] . It has been reported that miRNA target accessibility is a critical factor in determining miRNA function [56] . The targeted mRNA secondary structure and the sequence context surrounding miRNA-binding sites all influence the repressional function of miRNAs [57] , [58] , and, similar to miRNA, the secondary structure also plays an important role in regulating the function of lncRNA [59] , [60] . In our present study, RNAhybrid analysis reveals a healthy minimum free energy of hybridization between lncRNA APF and miR-188-3p of −26.2 kcal mol −1 . Thus, it is indicated that lncRNA APF is accessible to miR-188-3p and the interaction between lncRNA APF and miR-188-3p is effective. The function of lncRNAs remains scantly identified. Although current available experimental tools used to elucidate lncRNA mechanisms are limited, the accessibility of miRNA and lncRNA is an interesting and important research topic. We will further excavate and study the underlying rules that govern lncRNA–miRNA interaction in our future work, which might provide new candidates for an effective treatment of cardiac diseases. Cardiomyocytes culture and treatment Cardiomyocytes were isolated from male mice (1–2 days), which were obtained from Institute of Laboratory Animal Science of Chinese Academy of Medical Sciences (Beijing, China). In brief, after dissection hearts were washed and minced in HEPES-buffered saline solution. Tissues were then dispersed in a series of incubations at 37 °C in HEPES-buffered saline solution containing 1.2 mg ml −1 pancreatin and 0.14 mg ml −1 collagenase. Subsequent supernatants were collected and centrifuged at 200 g for 5 min. After centrifugation, cells were re-suspended in Dulbecco’s modified Eagle medium/F-12 (GIBCO) containing 5% heat-inactivated horse serum, 0.1 mM ascorbate, insulin-transferring-sodium selenite media supplement (Sigma, St Louis, MO), 100 U ml −1 penicillin, 100 μg ml −1 streptomycin and 0.1 mM bromodeoxyuridine. The dissociated cells were pre-plated at 37 °C for 1 h. The cells were then diluted to 1 × 10 6 cells ml −1 and plated in 10 μg ml −1 laminin-coated different culture dishes according to the specific experimental requirements. A/R was performed as follows. Cells were placed in an anoxic chamber with a water-saturated atmosphere comprising 5% CO 2 and 95% N 2 . After anoxia, the cells were subjected to reoxygenation (95% O 2 and 5% CO 2 ). Cell death assay Cell death was determined by Trypan Blue exclusion, and the numbers of Trypan Blue-positive and Trypan Blue-negative cells were counted on a haemocytometer. Adenoviral constructions and infection The mouse APF was synthesized by PCR using mouse cDNA as the template. The forward primer was 5′-AAATCTCTTTGAACAAGGTAAC-3′; the reverse primer was 5′-CCAAAGTCGGCTGAGTTTGCTCTTA-3′. Mouse ATG7 cDNA was from Origene. To produce mutated APF (APF-mut) and mutated ATG7 (ATG7-mut), the mutations were generated using QuikChange II XL Site-Directed Mutagenesis Kit (Stratagene). The adenoviruses harbouring the APF, APF-mut, ATG7-mut and β-galactosidase (β-gal) were constructed using the Adeno-XTM expression system (Clontech). The mouse APF RNA interference (siRNA) target sequence is 5′-TTGTGAGACTACCTCACTG-3′. A scramble form was used as a control, 5′-CGCTTCTCTAGCTAGTAGA-3′. The mouse ATG7 RNA interference (siRNA) target sequence is 5′-TGGTGACTCTGCTGGTCTG-3′. A scramble form was used as a control, 5′-TCGTGTCAGTTCTGGTGGC-3′. The adenoviruses harbouring APF siRNA, ATG7 siRNA and their scramble forms were constructed using the pSilencer adeno 1.0-CMV System (Ambion) according to the Kit’s instructions. All constructs were amplified in HEK293 cells. Western blot Immunoblot was performed as follows. The cells were lysed for 1 h at 4 °C in a lysis buffer (20 mmol l −1 Tris pH 7.5, 2 mmol l −1 EDTA, 3 mmol l −1 EGTA, 2 mmol l −1 dithiothreitol (DTT), 250 mmol l −1 sucrose, 0.1 mmol l −1 phenylmethylsulfonyl fluoride and 1% Triton X-100) containing a protease inhibitor cocktail. The samples were subjected to 12% sodium dodecyl sulfate–PAGE (SDS–PAGE) and transferred to nitrocellulose membranes. Equal protein loading was controlled by Ponceau Red staining of membranes. Blots were probed using the primary antibodies. The anti-ATG7 antibody (1:500, Abcam), anti-PCNA antibody (1:1,000, Santa Cruz Biotechnology), anti-Tubulin antibody (1:2,000, Abcam), anti-Beclin 1 antibody (1: 1,000, Abcam) and anti-LC3 antibody (1:500, Abcam) were used in this study. After four times washing with PBS, the horseradish peroxidase-conjugated secondary antibodies were added. Antigen–antibody complexes were visualized by enhanced chemiluminescence. Full-sized scans of western blots are provided in Supplementary Fig. 8 . Luciferase constructs and transfection ATG7 3′UTR was amplified by PCR. The forward primer was 5′-TGTCTGAAGCAAGCAACCACAG-3′. The reverse primer was 5′-GCTTGTTGCAGCATCTGTGTTA-3′. To produce mutated 3′UTR, the mutations were generated using QuikChange II XL Site-Directed Mutagenesis Kit (Stratagene). Wild type and mutated 3′UTRs were subcloned into the pGL3 vector (Promega) immediately downstream the coding region of luciferase gene. Mouse APF wild type (APF-wt) and the mutant derivative devoid of miR-188-3p binding site (APF-mut) were cloned downstream the coding region of luciferase gene. The forward primer was 5′-AAATCTCTTTGAACAAGGTAAC-3′; the reverse primer was 5′-CCAAAGTCGGCTGAGTTTGCTCTTA-3′. HEK293 cells or cardiomyocytes were infected with the indicated adenoviruses, then transfected with the indicated luciferase constructs as described in the corresponding figure legends. The transfection was performed using Lipofectamine 2000 (Invitrogen) according to the manufacturer’s instruction. The luciferase activity was analysed as we described elsewhere [61] . Quantitative reverse transcription-PCR Stem-loop reverse transcription-PCR (qRT-PCR) for mature miR-188-3p was performed on a CFX96 real-time PCR detection system (Bio-Rad). First, total RNA was extracted using Trizol reagent. After DNAse I (Takara, Japan) treatment, RNA was reverse transcribed with reverse transcriptase (ReverTra Ace, Toyobo) using the stem-loop RT primer, which is hybridized to miR-188-3p. Next, the RT products are quantified using SYBR Green real-time PCR. The levels of miR-188-3p analysed by qRT–PCR were normalized to that of U6. U6 primers were forward: 5′-GCTTCGGCAGCACATATACTAA-3′; reverse: 5′-AACGCTTCACGAATTTGCGT-3′. APFs were quantified using SYBR Green real-time PCR. The sequences of APF primers were forward: 5′-CTCCTCTATATTGTGTTCAAG-3′; reverse: 5′-GTGTTCATAAGGTAACCTGAA-3′. The results were standardized to control values of glyceraldehyde-3-phosphate dehydrogenase (GAPDH). GAPDH forward primer: 5′-TGTGTCCGTCGTGGATCTGA-3′; reverse: 5′-CCTGCTTCACCACCTTCTTGA-3′. The specificity of the PCR amplification was confirmed by agarose gel electrophoresis. Target protector preparation and transfection Target protector was designed to disrupt the interaction of specific miRNA–mRNA pairs. Target protector sequence is complementary to miR-188-3p-binding site in target ATG7. In brief, ATG7-TP miR-188-3p sequence is 5′-CTCCCATCCCTGGAACAGGGTGGCA-3′. ATG7-TP control sequence is 5′-CCTCTTACCTCAGTTACAATTTATA-3′. They were synthesized by Gene Tools, and transfected into the cells using the Endo-Porter kit (Gene Tools) according to the kit’s instructions. Absolute quantification using real-time RT-PCR We measured the absolute copy number using the standard curve method. The cDNA of APF was cloned into pcDNA 3.1 vector. The vector was linearized and generated sense RNA transcript using in vitro T7 promoter transcription system (Promega). After digested with RNAse-free DNAse and purification, the transcript was quantified on a spectrophotometer and converted to the number of copies using the following formula: Copy number μl −1 . The quantified RNA was used as the standard of APF. Synthetic miR-188-3p RNA was used as the standard of miR-188-3p. For detection of APF, the standard and total RNA were reverse transcribed with ReverTra Ace (Toyobo) using the reverse primer. The standard of miR-188-3p was reverse transcribed same as the endogenous miR-188-3p. The standard cDNA was serially diluted in nuclease-free water. Serial dilutions from 10 6 to 10 1 copies were used for standard in a final volume of 20 μl alongside a negative control (RNA) and a non-template control. The SYBR Premix Ex Taq II Kit (Takara) was used for amplification. Quantitative PCR was performed on a CFX96 real-time PCR detection system (Bio-Rad). Absolute quantification determines the actual copy numbers of target genes by relating the Ct value to a standard curve. The data were analysed by CFX96 software. The final data were expressed as the copy number per 10 pg of total RNA. Preparations of subcellular fractions Subcellular fractions were prepared as follows. The cells were washed twice with PBS and the pellets were suspended in 0.2 ml of buffer A (20 mmol l −1 HEPES pH 7.5, 10 mmol l −1 KCl, 1.5 mmol l −1 MgCl2, 1 mmol l −1 EGTA, 1 mmol l −1 EDTA, 1 mmol l −1 DTT, 0.1 mmol l −1 PMSF and 250 mmol l −1 sucrose) containing a protease inhibitor cocktail. The cells were homogenized by 12 strokes in a Dounce homogenizer. The homogenates were centrifuged twice at 750 g for 5 min at 4 °C to collect nuclei and debris. The supernatants were centrifuged at 10,000 g for 15 min at 4 °C to collect mitochondria-enriched heavy membrane pellet. The resulting supernatants were centrifuged to yield cytosolic fractions. Transfection of the antagomirs The chemically modified antagomirs complementary to miR-188-3p designed to inhibit endogenous miR-188-3p expression, and the antagomir-negative control (antagomir-NC) was obtained from GenePharma. The antagomir sequence was 5′-UGCAAACCCUGCAUGUGGGAG-3′. The antagomir-NC sequence was 5′-CAGUACUUUUGUGUAGUACAA-3′. Cells were transfected with the antagomirs or the antagomir-NC using Lipofectamine 2000 (Invitrogen) according to the manufacturer’s instruction. Pull-down assay with biotinylated DNA probe The biotinylated DNA probe complementary to APF was synthesized and dissolved in 500 μl of wash/binding buffer (0.5M NaCl, 20 mM Tris-HCl, pH 7.5, and 1 mM EDTA). The probes were incubated with streptavidin-coated magnetic beads (Sigma) at 25 °C for 2 h to generate probe-coated magnetic beads. Cardiomyocyte lysates were incubated with probe-coated beads, and after washing with the wash/binding buffer, the RNA complexes bound to the beads were eluted and extracted for northern blot analysis; APF pull-down probe, 5′-GAGATGGCAAAGGGGAACGCTCGATCC-3′; and random pull-down probe, 5′-TGATGTCTAGCGCTTGGGCTTTG-3′. Pull-down assay with biotinylated miRNA Cardiomyocytes were transfected with biotinylated miRNA (50 nM), harvested 48 h after transfection. The cells were washed with PBS followed by brief vortex, and incubated in a lysis buffer (20 mM Tris, pH 7.5, 200 mM NaCl, 2.5 mM MgCl2, 0.05% Igepal, 60 U ml −1 Superase-In (Ambion), 1 mM DTT, protease inhibitors (Roche)) on ice for 10 min. The lysates were precleared by centrifugation, and 50 μl of the sample was aliquoted for input. The remaining lysates were incubated with M-280 streptavidin magnetic beads (Sigma). To prevent non-specific binding of RNA and protein complexes, the beads were coated with RNase-free BSA and yeast tRNA (both from Sigma). The beads were incubated at 4 °C for 3 h, washed twice with ice-cold lysis buffer, three times with the low salt buffer (0.1%SDS, 1%Trition X-100, 2 mM EDTA, 20 mM Tris-HCl pH8.0 and 150 mM NaCl) and once with the high salt buffer (0.1%SDS, 1%Trition X-100, 2 mM EDTA, 20 mM Tris-HCl pH 8.0 and 500 mM NaCl). The bound RNAs were purified by Trizol for the analysis. Northern blot analysis The cell samples were collected and run on a 15% polyacrylamide-urea gel, transferred to positively charged nylon membranes (Millipore) followed by cross-linking through UV irradiation. The membranes were subjected to hybridization with 100 pmol 3′-digoxigenin (DIG)-labelled probes overnight at 42 °C. Probes were labelled with DIG using a 3′-End DIG Labelling Kit (Roche). The detection was performed using a DIG luminescent detection kit (MyLab) according to the manufacturer’s instructions. The probe sequence for miR-188-3p was 5′-TGCAAACCCTGCATGTGGGAG-3′. U6 was used as an internal control, and its probe sequence was 5′-GCTAATCTTCTCTGTATCGTTCC-3′. Transmission electron microscopy Conventional electron microscopy was performed as described previously [62] . In brief, cells were fixed with 2.5% glutaraldehyde and then postfixed with 1% osmium tetraoxide, dehydrated in a graded series of ethanol concentrations and embedded in Embed812 resin. The ultrathin sections were mounted on copper grids and then double-stained with uranyl acetate and lead citrate. The number of autophagic vacuoles was determined for a minimum of 100 cells. Heart ultrastructural analysis was also performed. The samples were examined and photographed with a FEI Tecnai spirit transmission electron microscope. Animal experiments Male adult C57BL/6 mice (8 weeks old) were obtained from Institute of Laboratory Animal Science of Chinese Academy of Medical Sciences (Beijing, China). All experiments were performed according to the protocols approved by the Animal Care Committee, Qingdao University. The animals we chose for experiments had similar body weight, and animals with normal physiological index during surgical experiments were used for statistical analysis. For intracoronary delivery of adenoviruses, the mice were anaesthetized and ventilated with a HX-300S animal ventilator. Entered into the chest through a small left anterior thoracotomy, the pericardial sac was then removed, and 2 × 10 10 m.o.i. adenoviruses of APF-siRNA, 2 × 10 11 m.o.i. adenoviruses of APF, 2 × 10 11 m.o.i. adenoviruses of APF-mut, 2 × 10 10 m.o.i. adenoviruses of ATG7-mut or 2 × 10 10 m.o.i. adenoviruses of ATG7-siRNA were injected with a catheter from the apex of the left ventricle into the aortic root while the aorta and pulmonary arteries were cross-clamped. The clamp was maintained for 20 s when the heart pumped against a closed system. After removal of air and blood, the chest was then closed and the mice were returned back to cage for recovery. Five days after the injection of adenoviruses, the mice were subjected to I/R surgery. For miR-188-3p mimics delivery, chemically modified mimics were 2′-OMe modified (GenePharma, Shanghai). The mice received on three consecutive days, intravenous injections of mimics and their controls at doses of 30 mg kg −1 body weight in a small volume (0.2 ml) per injection. The mice were then subjected to I/R surgery. For ATG7 target protector delivery, the target protectors were delivered to the mice by i.v. injection once daily for three consecutive days at 25 mg kg −1 and the mice were then subjected to I/R surgery. For I/R injury model, mice were subjected to 45 min ischaemia, then 3 h or 1 week reperfusion. We anaesthetized the animals, opened the chest and exposed the heart to identify the left anterior descending coronary artery (LAD). We passed a silk suture around the LAD at the inferior border of left auricle and occluded the artery by snaring with a vinyl tube through which the ligature had been passed. We occluded the coronary artery by pulling the snare tight and securing it with a haemostat. After 45 min of ischaemia, we released the ligature and reperfused the heart. The Sham-operated group experienced the same procedure except the snare was left untied. After 3 h of reperfusion, evans blue dye (1 ml of a 2.0% solution; Sigma-Aldrich) was injected into jugular vein into the heart for delineation of the ischaemic zone from the non-ischaemic zone. The heart was rapidly excised. The heart slices were incubated in 1.0% 2,3,5-triphenyltetrazolium chloride (Sigma-Aldrich) for 15 min at 37 °C for demarcation of the viable and nonviable myocardium within the risk zone. The staining was stopped by ice-cold sterile saline, and the slices were fixed in 10% neutral buffered formaldehyde and individually weighed. Both sides of each slice were photographed. The areas of infarction (INF) and risk zone were assessed with computer-assisted planimetry (NIH Image 1.57) by an observer blinded to the sample identity. The ratio of INF/risk zone was calculated. Echocardiographic assessment Transthoracic echocardiographic analysis was performed on mice after 1 week of the sham or I/R surgery. We obtained echocardiographic parameters including systolic left ventricular internal diameters (LVIDs) and diastolic left ventricular internal diameters (LVIDd). We calculated fractional shortening (FS) of left ventricular diameter as [(LVIDd—LVIDs)/LVIDd] × 100. After in vivo evaluation of cardiac function the mice were killed and the hearts were harvested, weighted and used for histological examination. Statistical analysis Data are expressed as the mean±s.e.m. of at least three independent experiments for each cellular experimental group and at least five independent experiments for each animal group. We evaluated the data with Student’s t test. We used a one-way analysis of variance for multiple comparisons. A value of P <0.05 was considered significant. How to cite this article: Wang, K. et al. APF lncRNA regulates autophagy and myocardial infarction by targeting miR-188-3p. Nat. Commun. 6:6779 doi: 10.1038/ncomms7779 (2015).